Bidecadal North Atlantic ocean circulation variability controlled by timing of volcanic eruptions While bidecadal climate variability has been evidenced in several North Atlantic paleoclimate records, its drivers remain poorly understood. Here we show that the subset of CMIP5 historical climate simulations that produce such bidecadal variability exhibits a robust synchronization, with a maximum in Atlantic Meridional Overturning Circulation (AMOC) 15 years after the 1963 Agung eruption. The mechanisms at play involve salinity advection from the Arctic and explain the timing of Great Salinity Anomalies observed in the 1970s and the 1990s. Simulations, as well as Greenland and Iceland paleoclimate records, indicate that coherent bidecadal cycles were excited following five Agung-like volcanic eruptions of the last millennium. Climate simulations and a conceptual model reveal that destructive interference caused by the Pinatubo 1991 eruption may have damped the observed decreasing trend of the AMOC in the 2000s. Our results imply a long-lasting climatic impact and predictability following the next Agung-like eruption. The Atlantic Meridional Overturning Circulation (AMOC) plays a key role in the meridional heat transport, and in heat and carbon storage in the ocean [1] . Changes in the AMOC affect surface oceanic conditions in the North Atlantic (salinity, temperature and sea level), with impacts on marine ecosystems and regional climate (for example, Greenland glaciers [2] ). Understanding the mechanisms driving AMOC decadal variability is therefore critical for climate predictability, particularly in the Northern Hemisphere [3] , [4] , [5] . In response to increased greenhouse gas concentrations, climate models project a gradual AMOC slowdown during the 21st century [6] , [7] . AMOC strength has only recently been monitored through observation networks. Existing data sets do not reveal a strong trend in the 2000s [8] , [9] , although a declining tendency appears from the early 2010s [10] , [11] . This is also supported by ocean reanalyses [12] , [13] , which depict an AMOC maximum in the 1990s at subpolar latitudes, followed by a decrease and stabilization in the 2000s. Beyond direct information on AMOC, North Atlantic observations [14] , [15] and proxy records indicate a 20-year preferential variability in this region in the atmosphere [16] , sea ice [17] and the ocean [18] , [19] . Such variability can be associated with the dynamics of subpolar gyre, whose characteristic decadal timescales are associated with advection processes and the size of the gyre [20] , [21] . Indeed, such advective processes have been observed during Great Salinity Anomaly (GSA) events [22] , [23] , [24] . For instance, a salinity anomaly was first identified in the Nordic Seas in 1968, and then detected in the Labrador Sea around 1971. This anomaly was monitored along its propagation within the subpolar gyre during the following 7 years, and it reached the eastern part of the Nordic Seas in 1978 (ref. 22 ). Explosive volcanic eruptions have a short-lived but strong radiative impact through the loading of a large amount of sulphate aerosols into the stratosphere, which leads to a cooling of the Earth’s surface during the 2–3 years following the onset of the eruption [25] , [26] . Moreover, the volcanic sulphate aerosol injection causes a significant stratospheric warming in the tropical band due to long-wave heat absorption. The subsequent strengthening of the meridional atmospheric temperature gradient leads to intensified zonal winds and jets through thermal wind balance. As a result, observations show that volcanic eruptions trigger dynamical changes [27] , [28] , with a tendency towards a positive phase of the winter North Atlantic Oscillation (NAO, first mode of atmospheric variability in the north Atlantic sector [29] ) during the few years following the eruption [27] , [30] , [31] . This dynamical mechanism is not well represented in most climate simulations, at least partly due to a too coarse vertical resolution of their atmospheric model component [27] . In addition, climate model analysis suggests that the volcanic-driven, short-lived cooling of the upper ocean can induce longer-lived changes on North Atlantic climate, notably through its influence on the AMOC [32] , [33] , [34] . The robustness of the mechanisms at play have, however, been challenged by differences in the simulated timing and response, suggesting a sensitivity of the results to the model used or to the prescribed volcanic forcing. Oceanographic data have not yet been used to evaluate the exact oceanic processes at play. Here we evaluate the potential impact of moderate explosive volcanic eruptions (similar to Agung or Pinatubo) on the North Atlantic bidecadal preferential variability. For this purpose, we use available outputs from different climate models using the Coupled Model Intercomparison Project Phase 5 (CMIP5) database [35] complemented by additional simulations performed using one model, and in situ recent oceanic observations as well as longer paleoclimate proxy records of the last millennium. We find that moderate volcanic eruptions may reset a 20-year intrinsic variability mode in the North Atlantic both in model simulations as well as in the data analyzed, leading to interference patterns over the recent period and in the near future. Analysis of the CMIP5 database We investigate the mechanisms involved in bidecadal North Atlantic and AMOC variations and reduced AMOC variability around the trend during the 2000s using CMIP5 simulations and sensitivity tests conducted specifically with the IPSL-CM5A-LR model [36] . Historical climate simulations (1870–2005) driven by natural and anthropogenic forcing archived in the CMIP5 database exhibit a large spread in the simulated AMOC at 48°N ( Fig. 1a ). 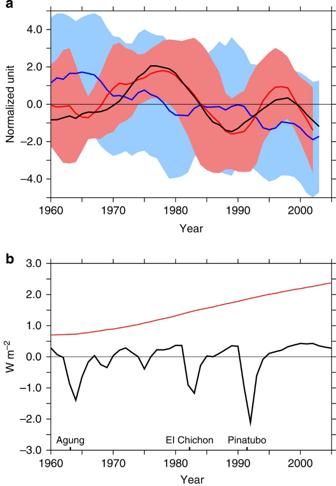Figure 1: Simulated AMOC changes and radiative external forcing. (a) Variations of the AMOC maximum at 48°N over the period 1960–2005 for the ensemble of five historical simulations performed with the IPSL-CM5A-LR model (black); for the Bi-Dec ensemble excluding the IPSL-CM5A-LR simulation (subset of eight CMIP5 models, which also exhibit variability in the 10–30 years spectral band, in red, see Methods,Supplementary Table 1andSupplementary Fig. 1); for the ensemble mean of the 10 other CMIP5 historical simulations (in blue). The standard deviation (s.d.) of the two CMIP5 ensembles is shown with the red and blue envelopes. All the AMOC indices have been normalized with the s.d. of the detrended time series over the period 1850–2005. (b) External radiative forcing (in W m−2) computed in the IPSL-CM5A-LR historical simulation. The black curve is the natural forcing including solar and volcanic eruptions and the red curve represents the anthropogenic forcing including greenhouse gas changes and the anthropogenic aerosols effects. A 5-year running mean has been applied to all time series froma. Out of 19 available model simulations, we select the subset of 9 (8+IPSL-CM5A-LR called ‘Bi-Dec’ ensemble) which exhibit peaks of spectral energy in the 10–30 years band for either the historical or the pre-industrial simulations ( Supplementary Table 1 , Supplementary Figs 1 and 2 ). Because this frequency peak is clearly evidenced in North Atlantic proxy records [16] , [17] , [18] , we expect these selected models to potentially capture the actual variability pattern. In the IPSL-CM5A-LR model, strong 20-year variability in the North Atlantic is related to the time scale of temperature and salinity advection in the subpolar gyre, with salinity anomalies driving convection and deep ocean circulation [20] . The Bi-Dec ensemble shows coherent AMOC variability at 48°N (with an ensemble correlation coefficient of 0.64, significant at the 99% level), not seen in the ensemble of the remaining CMIP5 historical runs ( Fig. 1a and Supplementary Fig. 2 ). More precisely, the Bi-Dec members systematically exhibit an AMOC maximum in the late 1970s. This consistent timing among them strongly suggests the response to a common external forcing. Earlier modelling studies have indeed shown intensified AMOC about a decade after strong volcanic eruptions [26] , [32] , [33] , the lag reflecting the time required for the advection of cold anomalies from the subtropics to high latitudes, and for the response of the AMOC to changes in atmospheric momentum forcing. Here we suggest that the 1963 Agung eruption ( Fig. 1b ) has reset bidecadal variability in the eight CMIP5 simulations, leading to a first AMOC maximum about 15 years later (late 1970s). A second (weaker) simulated maximum occurs in the 1990s, corresponding to a secondary peak from the 20-year mode ( Fig. 1 ). The same features are reproduced in a five-member ensemble of historical simulations from the IPSL-CM5A-LR model [13] . Figure 1: Simulated AMOC changes and radiative external forcing. ( a ) Variations of the AMOC maximum at 48°N over the period 1960–2005 for the ensemble of five historical simulations performed with the IPSL-CM5A-LR model (black); for the Bi-Dec ensemble excluding the IPSL-CM5A-LR simulation (subset of eight CMIP5 models, which also exhibit variability in the 10–30 years spectral band, in red, see Methods, Supplementary Table 1 and Supplementary Fig. 1 ); for the ensemble mean of the 10 other CMIP5 historical simulations (in blue). The standard deviation (s.d.) of the two CMIP5 ensembles is shown with the red and blue envelopes. All the AMOC indices have been normalized with the s.d. of the detrended time series over the period 1850–2005. ( b ) External radiative forcing (in W m −2 ) computed in the IPSL-CM5A-LR historical simulation. The black curve is the natural forcing including solar and volcanic eruptions and the red curve represents the anthropogenic forcing including greenhouse gas changes and the anthropogenic aerosols effects. A 5-year running mean has been applied to all time series from a . Full size image We do not expect such coherent variability to arise from the gradual long-term anthropogenic forcing. While solar forcing has been shown to influence ocean circulation variability in a climate model [37] , solar forcing had a weak radiative amplitude of variability compared with volcanic eruptions, especially during the second half of the 20 th century. We therefore propose that the coherent signal identified in the simulations has been triggered by the 1963 Agung volcanic eruption. Such large volcanic eruptions are indeed known to strongly cool the surface of the North Atlantic subpolar gyre and the Nordic Seas [32] , [34] , [38] (see for example, Supplementary Fig. 3 ). The bidecadal time scale of the subsequent dynamical adjustment to temperature anomalies involves the advection of temperature and salinity anomalies [15] (for example, GSAs) or baroclinic instabilities leading to large-scale baroclinic Rossby waves [21] , [39] , [40] , strongly constrained by the size of the subpolar basin, and interactions with sea ice and atmospheric circulation. The specific processes accounting for the bidecadal variability may differ in the different climate models [21] . In the following, we will focus on one specific climate model (IPSL-CM5A-LR), for which the mechanisms underlying this variability [20] , [41] as well as its response to recent volcanic eruptions have been recently investigated in depth [15] . Simulations over the historical period, the last millennium, as well as additional sensitivity simulations performed with this model are discussed and compared with in situ oceanic data as well as proxy records. Comparison with recent oceanic data Recent AMOC variability cannot be assessed in the short 2004-to-present observational record [8] , [11] . An alternative strategy is to use salinity observations, which exhibit large and well-documented variability in the North Atlantic, most notably as GSA. These GSAs occurred in the 1970, 1980 and 1990s ( Fig. 2b ). The current understanding is that the 1980s event was forced by the atmospheric circulation, while the 1970 and 1990s events are associated with Arctic Ocean variability via the East Greenland Current (EGC) [22] , [24] . Changes in salinity play a crucial role in the stability of the water column. They can drive changes in oceanic convection, which is directly related to AMOC variability. Here we use a combination of North Atlantic surface and subsurface salinity observational data sets (spanning years 1949–2010): a reconstruction of surface salinity in the eastern subpolar gyre [42] , a new compilation of salinity data over a region enclosing large part of the Labrador Sea and reaching down to 300 m (compiled from the Bedford Institute of Oceanography website, see for example, Methods) and the global EN3 (ref. 43 ) data set ( Fig. 2b ). These data sets are compared with the IPSL-CM5A-LR ensemble of historical simulations. 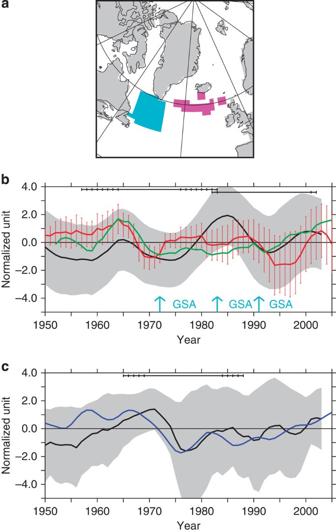Figure 2: Observed and simulated changes in salinity. (a) Location of the two key regions (Labrador Sea and subpolar gyre) studied here. (b)In situsalinity data from the Labrador Sea averaged over the cyan region down to 300 m compiled from the Bedford Institute (see for example, Methods, red line, with vertical line representing 2-s.d. errors) and from EN3 (ref.43) (green) observational data sets. (c) Sea Surface Salinity fromin situdata42(in blue) averaged over the eastern subpolar gyre (magenta region). Inb,c, the 5-member ensemble mean outputs from historical simulations using IPSL-CM5A-LR are also displayed (black, mean value; grey shaded, s.d. envelope). The horizontal black lines at the top ofb,cdelimit the 20-year sliding windows for which significant correlation is detected (at the 95% confidence level) between the simulations and the observations (using the Bedford Institute data only inb. A 5-year running mean has been applied to all time series. Figure 2: Observed and simulated changes in salinity. ( a ) Location of the two key regions (Labrador Sea and subpolar gyre) studied here. ( b ) In situ salinity data from the Labrador Sea averaged over the cyan region down to 300 m compiled from the Bedford Institute (see for example, Methods, red line, with vertical line representing 2-s.d. errors) and from EN3 (ref. 43 ) (green) observational data sets. ( c ) Sea Surface Salinity from in situ data [42] (in blue) averaged over the eastern subpolar gyre (magenta region). In b , c , the 5-member ensemble mean outputs from historical simulations using IPSL-CM5A-LR are also displayed (black, mean value; grey shaded, s.d. envelope). The horizontal black lines at the top of b , c delimit the 20-year sliding windows for which significant correlation is detected (at the 95% confidence level) between the simulations and the observations (using the Bedford Institute data only in b . A 5-year running mean has been applied to all time series. Full size image Figure 2 shows that the IPSL-CM5A-LR simulations capture the observed 1970 and 1990s GSAs in the Labrador Sea and Eastern subpolar gyre. In this model, an increase in the EGC leads to a decreased salinity in the Labrador Sea, followed by AMOC variations about 10 years later [20] . Detailed analyses [15] have shown that changes in salinity simulated by the IPSL-CM5A-LR in the 1970s are a dynamical response to the Agung eruption. Here we conclude that the Agung eruption has excited the bidecadal mode of the North Atlantic in both observations and simulations, explaining not only the GSA of the 1970s but also the subsequent GSA of the 1990s. During both the 1970 and 1990s GSA events, salinity anomalies are associated with local temperature minima in the observations ( Supplementary Fig. 4 ), consistently with the mechanism at play in the IPSL-CM5A-LR model [20] . This agreement between model and observations can be extended to the Bi-Dec ensemble. Indeed similar GSAs as the observed ones in the 1970 and 1990s are found in this ensemble mean as in the observations in the Labrador Sea both for salinity and temperature ( Supplementary Fig. 5 ). The large spread in the ensemble also shows that the exact locations of the anomalies and of the processes at play are model dependent. It has been suggested that the GSA encountered in the 1980s, which is clearly weaker than the two others in the Bedford compilation ( Fig. 2 ), and is not depicted by the IPSL-CM5A-LR historical simulations, may have a different origin [22] . This specific GSA was indeed associated with extremely severe winters of the early 1980s, with a possible contribution of the Arctic freshwater outflow via the Canadian Archipelago [22] . If this GSA was indeed driven by extreme stochastic atmospheric processes, this might explain the fact that it is not captured in the historical simulations, as well as the smaller amplitude and depth of this event as compared with the two other GSAs ( Fig. 2b ). We therefore hypothesize that this smaller GSA may not have strongly affected convection in the subpolar gyre, with therefore a very weak signature on the AMOC variability, in contrast with the two other GSA. This is however not fully supported by the fingerprint of the 1980s GSA in the EN3 data set, challenging this interpretation. Last millennium perspective To further assess the validity of the excitation of bidecadal variations by volcanic eruptions, we investigate two high-resolution proxy records and a new IPSL-CM5A-LR simulation spanning the last millennium, which includes several earlier Agung-like volcanic eruptions. This simulation also exhibits a clear spectral peak at the 20-year time scale for the 48°N AMOC variability ( Supplementary Fig. 6 ). The first proxy record is an updated compilation of six annually resolved δ 18 O reconstructions from Greenland ice cores (see Methods and Supplementary Fig. 1 ). From an Empirical Orthogonal Function (EOF) analysis, their leading common signal is extracted, corresponding to a monopole that exhibits preferential variability at a 20-year time scale ( Fig. 3 ), coherent with earlier ice core composites [3] . This data set is highly correlated with North Atlantic Sea Surface Temperature (SST) as shown by the regression of HadISST data [44] on the principal component (PC) of the first EOF from the ice cores for the period 1850–1973 ( Fig. 4 ). Significant correlation is indeed found in the Atlantic, approximately from the equator to the Nordic Seas, a spatial pattern that is reminiscent of the Atlantic Multidecadal Oscillation [45] (AMO). The response is especially large in the North Atlantic ( Fig. 4a ). To test this relationship on a longer time scale, we use a gridded SST reconstruction [46] and perform the same regression analysis for the period 1000–1850. Again, significant correlation is mainly found in the Atlantic basin north of the equator ( Fig. 4b ). Although this second result should be taken with caution, given that the SST reconstruction is based on a multi-proxy approach, also including Greenland ice core data, we argue that the ice core compilation provides an annually resolved record of bidecadal North Atlantic surface temperature variability. Such bidecadal timescales are usually filtered out in AMO reconstructions [46] , [47] , which indeed act as low pass filters and stress multidecadal variability. We thus interpret this first EOF of Greenland ice cores as a proxy for North Atlantic SST variations in line with a former hypothesis linking a stack of Greenland ice cores with surrounding SST [48] . 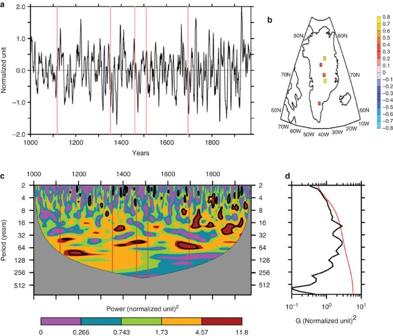Figure 3: Bidecadal variability in Greenland ice core data. (a) Principal component time series (with a 5-year running mean) associated with (b) the first EOF of the δ18O data from six annually resolved Greenland ice cores, computed over the period 1000–1973 (see for example, Methods). (c) Wavelet analysis of the time series shown inabut without any filtering. The region significant at the 95% level are marked using bold contours. (d) Power spectrum of the time series in black compared with an AR1 signal shown in red. Ina,c, the vertical red bars stand for the onset of the five eruptions selected over the last millennium. Figure 3: Bidecadal variability in Greenland ice core data. ( a ) Principal component time series (with a 5-year running mean) associated with ( b ) the first EOF of the δ 18 O data from six annually resolved Greenland ice cores, computed over the period 1000–1973 (see for example, Methods). ( c ) Wavelet analysis of the time series shown in a but without any filtering. The region significant at the 95% level are marked using bold contours. ( d ) Power spectrum of the time series in black compared with an AR1 signal shown in red. In a , c , the vertical red bars stand for the onset of the five eruptions selected over the last millennium. 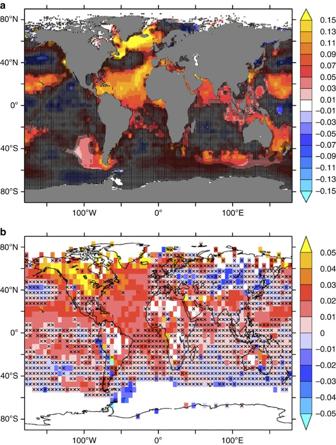Figure 4: Regression of the principal component of the Greenland ice core δ18O with sea surface temperature data sets. (a) For the period 1870–1974 with SST data from HadISST44and (b) over the period 1000–1850 with gridded surface temperature reconstructions46. The non-significant zones for the regression at 95% level are marked with a black cross. Full size image Figure 4: Regression of the principal component of the Greenland ice core δ 18 O with sea surface temperature data sets. ( a ) For the period 1870–1974 with SST data from HadISST [44] and ( b ) over the period 1000–1850 with gridded surface temperature reconstructions [46] . The non-significant zones for the regression at 95% level are marked with a black cross. Full size image The second proxy record corresponds to growth increments from the bivalve Arctica islandica collected north of Iceland [49] , also annually resolved. These bivalve data are not an unequivocal proxy for SST as they also depend on other factors, notably the nutrient supply [49] . The latter depends itself on vertical movements that can be related to AMOC variations, notably through convection processes which can help deep ocean nutrients to come to the surface [50] . For instance, in the isopycnal layered ESM2G Earth System model, strong inter-decadal changes in surface salinity associated with changes in AMOC produce spatially heterogeneous variability in convection, nutrients supply and thus diatom biomass [44] . As the IPSL-CM5A-LR model includes a bio-geochemical component [36] , [51] , we use it to test this hypothesis through a pseudo-proxy approach [52] . In particular, we analyze the link between nutrient concentrations (PO 4 , NO 3 , Si and Fe) and the 48°N AMOC index in the last millennium simulation. In this case, silicate and iron in the Nordic Seas are the main limiting nutrients for phytoplankton growth (not shown) and therefore expected to be also the limiting nutrients for bivalve growth, motivating a focus on these nutrients. Around Iceland, the simulated nutrients supply is significantly correlated with the simulated variations in 48°N AMOC, the latter leading the former by 1–3 years ( Fig. 5a ). We argue here that this relationship arises from changes in convection in the Nordic Seas, which precedes AMOC changes by 1–4 years [20] and changes in nutrient supplies around Iceland by 2–5 years in our model ( Fig. 5c ). This last lag can be explained by the upwelling of nutrients stored at depth by vertical currents associated with convection, and a subsequent period of a few years to export these nutrients from the convection sites towards north Iceland. Based on the hypothesis that the nutrient supply to Iceland is the limiting factor for the growth of the bivalve A. islandica , we therefore use growth increment records as a proxy of the subpolar AMOC, with a response lag of 1–3 years. 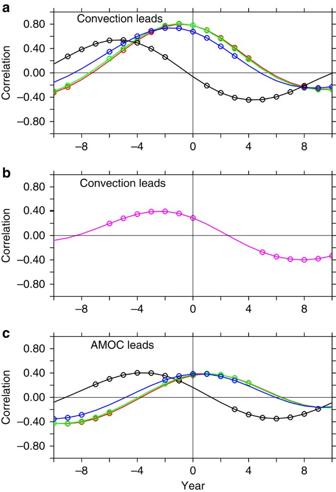Figure 5: Phase relationship between key variables of the last millennium IPSL-CM5A-LR simulation. Cross-correlation coefficients (y-axis) computed over the whole length of the last millennium simulation (850–1850) for different time lags (x-axis), (a) mixed layer depth in the Nordic Seas (an indicator of convection) and nutrient concentration north of Iceland, averaged between 50 and 150 m, where the bivalves are located. (b) Cross-correlation between mixed layer depth in the Nordic Seas and 48°N AMOC. (c) Same asbexcept that mixed layer depth in the Nordic Seas is replaced by 48°N AMOC. Ina,c, different colours are used to represent different nutrients (red, NO3; green, PO4; blue, Si and black, Fe). Correlation coefficients which are significant using a 95% confidence level Studentt-test (where degrees of freedom account for data autocorrelation70) are highlighted with circles. Figure 5: Phase relationship between key variables of the last millennium IPSL-CM5A-LR simulation. Cross-correlation coefficients ( y -axis) computed over the whole length of the last millennium simulation (850–1850) for different time lags ( x -axis), ( a ) mixed layer depth in the Nordic Seas (an indicator of convection) and nutrient concentration north of Iceland, averaged between 50 and 150 m, where the bivalves are located. ( b ) Cross-correlation between mixed layer depth in the Nordic Seas and 48°N AMOC. ( c ) Same as b except that mixed layer depth in the Nordic Seas is replaced by 48°N AMOC. In a , c , different colours are used to represent different nutrients (red, NO 3 ; green, PO 4 ; blue, Si and black, Fe). Correlation coefficients which are significant using a 95% confidence level Student t -test (where degrees of freedom account for data autocorrelation [70] ) are highlighted with circles. Full size image Using estimates of past volcanic radiative forcing [53] , we identify volcanic eruptions with a radiative forcing ranging between one to one and a half times the amplitude of the 1963 Agung eruption (Pinatubo being 1.4 times Agung in terms of global radiative forcing used in IPSL-CM5A-LR, see for example, Methods). To avoid any interference from successive events (see below), we retain only those not followed within 40 years by eruptions larger than 1.5 Agung. Only five of all the eruptions recorded over the last 1,000 years meet these two criteria (onset of the eruption in 1118, 1352, 1460, 1511, 1695, see for example, Supplementary Fig. 7 ). We first compare the simulated AMOC variations following these five eruptions with the Icelandic bivalve data. They exhibit a maximum both around 15 and 35 years following the eruptions ( Fig. 6a,b ). The slight shift that is found between the 48°N AMOC from the model and the bivalve observations [49] is consistent with the 3-year lag found in Fig. 5 . Indeed the 3-year lagged correlation between the model AMOC and the bivalve data ensemble means reaches 0.66 ( p -value <0.1 see for example, Supplementary Fig. 8a ). 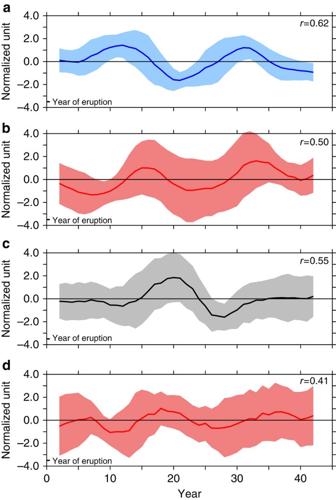Figure 6: Response to five Agung-like eruptions of the last millennium in reconstructions and IPSL-CM5-LR simulations. Time series of the composite formed by the ensemble of the five members for five Agung-like eruptions (taking place in 1118, 1352, 1460, 1511, 1695) over the last millennium identified through the same volcanic forcing reconstruction used in last millennium simulation53: (a) Simulated AMOC maximum at 48°N, (b) Growth increments in the bivalveArctica islandica49, (c) Simulated North Atlantic SST between 25 and 55°N, (d) first principal component of six yearly Greenland δ18O ice core reconstructions. The ensemble correlation between the five individual time series following the respective eruptions is shown for each index in top right of each panel. A 5-year running mean has been applied to all time series. Data have been standardized and expressed in normalized units. The average of the response following the five eruptions is shown with lines, and the envelope of the response is displayed through the shading around these lines. Figure 6: Response to five Agung-like eruptions of the last millennium in reconstructions and IPSL-CM5-LR simulations. Time series of the composite formed by the ensemble of the five members for five Agung-like eruptions (taking place in 1118, 1352, 1460, 1511, 1695) over the last millennium identified through the same volcanic forcing reconstruction used in last millennium simulation [53] : ( a ) Simulated AMOC maximum at 48°N, ( b ) Growth increments in the bivalve Arctica islandica [49] , ( c ) Simulated North Atlantic SST between 25 and 55°N, ( d ) first principal component of six yearly Greenland δ 18 O ice core reconstructions. The ensemble correlation between the five individual time series following the respective eruptions is shown for each index in top right of each panel. A 5-year running mean has been applied to all time series. Data have been standardized and expressed in normalized units. The average of the response following the five eruptions is shown with lines, and the envelope of the response is displayed through the shading around these lines. Full size image We then compare the simulated SST variations in the North Atlantic to the Greenland ice core data. They both exhibit coherent warming around 20 and 40 years after the eruptions ( Fig. 6c,d and Supplementary Fig. 8b ). The lag between AMOC and North Atlantic SST changes is attributed to a lagged accumulation of warm waters in the North Atlantic when the circulation accelerates [41] ( Supplementary Fig. 9 ) and is consistent with the results of other climate models [54] . Altogether, these results for five different Agung-type eruptions of the last millennium support the mechanism by which Agung-like volcanoes reset the 20-year AMOC variability. 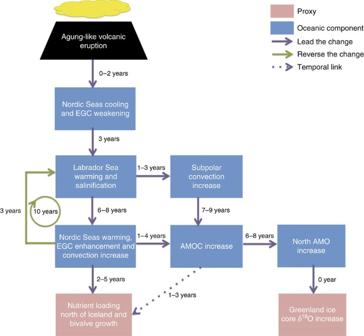Figure 7: Scheme summarizing the main processes at play in the North Atlantic response to volcanic eruptions. Blue boxes depict oceanic processes and red boxes depict the proxies considered here. Purple arrows represent causality links together with the associated time lags in years. Dotted arrows only depict a temporal link, with no direct interaction. The green arrow represents the delayed negative feedback that triggers the reversal phase of the 20-year cycle. Figure 7 summarizes the different processes proposed here as well as the time lags between them, including the proxy records analyzed. Figure 7: Scheme summarizing the main processes at play in the North Atlantic response to volcanic eruptions. Blue boxes depict oceanic processes and red boxes depict the proxies considered here. Purple arrows represent causality links together with the associated time lags in years. Dotted arrows only depict a temporal link, with no direct interaction. The green arrow represents the delayed negative feedback that triggers the reversal phase of the 20-year cycle. Full size image Interference pattern The implications of this oceanic response to moderate volcanoes like Agung or Pinatubo over the most recent 30-year period and the very near future are now investigated. Indeed, the Agung eruption was followed by the El Chichon eruption 19 years after and the Pinatubo eruption 28 years later. While the timing of El Chichon may have led to a constructive interference with the Agung-excited 20-year cycle, we make the hypothesis that the Pinatubo eruption interfered destructively; thereby explaining the damped observed and simulated AMOC variability in the 2000s. This hypothesis is tested using a five-member ensemble of IPSL-CM5A-LR starting in 1991 and using the same forcings as in the historical simulations but without the Pinatubo eruption. This ‘no Pinatubo’ sensitivity ensemble deviates from the historical ensemble ( Fig. 8a ) and exhibits much stronger practically bidecadal variability, with a minimum around 2010, a maximum in 2015 and a new minimum in 2025–2030. By contrast, the historical ensemble does not exhibit any remarkable decadal AMOC excursions from 2005 to 2030. Although the signal-to-noise ratio remains small and leads to an overlap of the s.d. envelopes of the two ensembles ( Supplementary Fig. 10 ), this sensitivity test confirms that the Pinatubo eruption induced a suppression of the bidecadal AMOC variability in the model. The simulated regular AMOC weakening in the 2010s after the Pinatubo eruption is consistent with the RAPID array observations [8] , [11] and with oceanic reanalyses [12] ( Fig. 8 ). 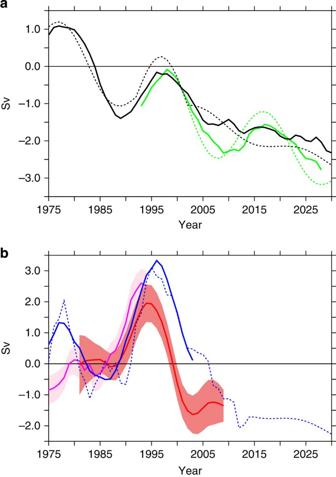Figure 8: Recent AMOC and projected change. (a) Simulated AMOC anomalies at 48°N in historical IPSL-CM5A-LR simulations (black), and in the sensitivity tests performed without taking into account the Pinatubo eruption (green). Results of the corresponding conceptual model (SI) are shown in dotted lines. (b) Estimates of AMOC at 45°N (1979–1988) based on hydrographic data13(pink curve) and ensemble mean of the AMOC maximum at 45°N from 12 ocean reanalyses12(red). This ensemble mean has been rescaled by a factor √12, to correct for the loss of variance caused by averaging different ocean models with different data assimilation. The five-member ensemble average of IPSL-CM5A-LR simulations nudged towards observed SST anomalies14is shown in blue. The dashed blue curve is the associated conceptual model including NAO variation (Methods). A 5-year running mean has been applied to all time series. Figure 8: Recent AMOC and projected change. ( a ) Simulated AMOC anomalies at 48°N in historical IPSL-CM5A-LR simulations (black), and in the sensitivity tests performed without taking into account the Pinatubo eruption (green). Results of the corresponding conceptual model (SI) are shown in dotted lines. ( b ) Estimates of AMOC at 45°N (1979–1988) based on hydrographic data [13] (pink curve) and ensemble mean of the AMOC maximum at 45°N from 12 ocean reanalyses [12] (red). This ensemble mean has been rescaled by a factor √12, to correct for the loss of variance caused by averaging different ocean models with different data assimilation. The five-member ensemble average of IPSL-CM5A-LR simulations nudged towards observed SST anomalies [14] is shown in blue. The dashed blue curve is the associated conceptual model including NAO variation (Methods). A 5-year running mean has been applied to all time series. Full size image This interference pattern from successive volcanoes can be captured by a simple conceptual model ( Fig. 9b ), which takes into account the timing of large volcanic eruptions that excited bidecadal oscillations over the last 60 years, assuming a constant response time, together with a long-term weakening trend [6] (see Methods). This conceptual model successfully reproduces the main features of the interference theory developed here, and closely follows the IPSL-CM5A-LR simulations with and without Pinatubo ( Fig. 8 ). However, neither the forced simulations nor this conceptual model are able to produce the rapid AMOC increase identified in the early 1990s in a few AMOC reconstructions [12] , [13] ( Fig. 8b ). It has been suggested that this specific shift is linked with internal atmospheric variability and 5-year-earlier changes in the NAO, which affected North Atlantic SST and therefore the decadal variability of the AMOC [3] , [55] , [56] . Indeed, climate simulations nudged towards observed SST anomalies performed using IPSL-CM5A-LR do produce a strong AMOC enhancement in the late 1990s that can be attributed to a NAO positive phase a few years earlier [15] ( Fig. 8 ). Similarly, implementing additional NAO variations in the conceptual model with a 5-year lagged response of the ocean (see Methods) reproduces most of the observed variability ( Fig. 8b ) as well as the very recent weakening over the last few years [10] . 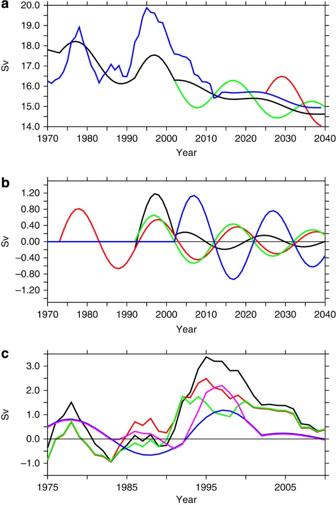Figure 9: Time evolution of the AMOC as computed by different conceptual models (described in Methods). (a) Different conceptual models with two (green) or three (black) volcanoes and with the NAO included (blue). For the future, when no NAO information is available, we take a null NAO phase. This allows illustration of the impact of an eruption in 2015 as shown in red. All the conceptual models include a long-term decreasing trend due to global warming (GW). (b) Decomposition of the impact of each volcano, Agung (in red), El Chichon (in green), Pinatubo (in blue) and the sum of the three (in black). (c) AMOC at 48°N from the different conceptual models, including or not including NAO variations following volcanic eruptions (see Methods). This decomposition allows estimation of the part of variance of the AMOC resulting from volcanic forcing and/or NAO, as compared with the total variance induced by volcanoes and NAO (black curve, 100% of the total variance). The red curve shows the calculation over the years 1975–2010 result when accounting for NAO (57% of the total variance), while the calculation accounting for NAO with the exception of the 3 years following each volcanic eruption is shown in green (44% of the total variance). The blue curve shows the bidecadal mode excitation by the volcanoes only (20% of the total variance), while the magenta curve shows the calculation when accounting for the impact of volcanoes plus the effect of the NAO in the 3 years following each eruption (30% of the total variance). Figure 9: Time evolution of the AMOC as computed by different conceptual models (described in Methods). ( a ) Different conceptual models with two (green) or three (black) volcanoes and with the NAO included (blue). For the future, when no NAO information is available, we take a null NAO phase. This allows illustration of the impact of an eruption in 2015 as shown in red. All the conceptual models include a long-term decreasing trend due to global warming (GW). ( b ) Decomposition of the impact of each volcano, Agung (in red), El Chichon (in green), Pinatubo (in blue) and the sum of the three (in black). ( c ) AMOC at 48°N from the different conceptual models, including or not including NAO variations following volcanic eruptions (see Methods). This decomposition allows estimation of the part of variance of the AMOC resulting from volcanic forcing and/or NAO, as compared with the total variance induced by volcanoes and NAO (black curve, 100% of the total variance). The red curve shows the calculation over the years 1975–2010 result when accounting for NAO (57% of the total variance), while the calculation accounting for NAO with the exception of the 3 years following each volcanic eruption is shown in green (44% of the total variance). The blue curve shows the bidecadal mode excitation by the volcanoes only (20% of the total variance), while the magenta curve shows the calculation when accounting for the impact of volcanoes plus the effect of the NAO in the 3 years following each eruption (30% of the total variance). Full size image For the 1975–2010 period, the conceptual model allows the relative importance of the response to volcanoes and to the NAO to be distinguished (see Methods). The NAO-induced AMOC variations account for 57% of the total AMOC variance, while 20% of the AMOC variance is due to excitation of the AMOC 15 years after volcanic eruptions, as a damped eigen mode (see for example, Fig. 9c ). The sum of the variance from this decomposition into two components does not equal 100%, indicating that there exists covariance between the components. This simple approach does not account for the potential impact of volcanoes on the NAO. While a strong positive NAO occurred in the 2–3 years following the Pinatubo eruption [28] , [30] , this is not a systematic response to all eruptions [57] . For instance, the winter following the Agung eruption had a negative NAO phase. This different response may arise from the intrinsic chaotic nature of the NAO, for which internal oscillations produce a large amount of noise, which can therefore mask a volcanic-forced signal. To address this issue, we repeat our analysis removing the NAO signature of the three winters following the three main volcanic eruptions considered. In the conceptual model, the fraction of AMOC variance explained by the response to volcanic forcing in 1975–2010 now increases to 30%, while NAO-only (without considering the three winters following eruptions) accounts for 44% of the variance (see for example, Fig. 9c and Methods). Once again, we note some covariance within this decomposition leading to a sum lower than 100%. We have shown here multiple lines of evidence supporting the long-lasting impact of moderate (Agung-size) volcanic eruptions on ocean circulation in the North Atlantic. The timing of subsequent volcanic eruptions can lead to constructive (for example, Agung and El Chichon) or destructive interferences (for example, Agung and Pinatubo) to force internal modes of ocean variability. In the IPSL-CM5A-LR model, the underlying mechanism is related to the build-up and advection of salinity anomalies near the Labrador region, and its subsequent effect on North Atlantic convection. Moderate volcanoes increase the sea-ice cover in the Nordic Seas, thus reducing the export of freshwater through the Denmark Strait and leading to anomalous positive anomalies in the Labrador region, explaining the observed GSAs of the 1970 and 1990s. While the exact processes at play may be model dependent, the coherence of the Bi-Dec model responses suggest a key role for the propagation of salinity and temperature anomalies as observed during GSA events. The exact path and pattern for this propagation may vary among the models that exhibit bidecadal AMOC variability, including, for example, the strength of the amplifying mechanisms through sea ice and atmosphere interactions, clearly depicted by the IPSL-CM5A-LR model. Further intercomparisons of the precise mechanisms at play within the different models are needed to understand this potential diversity. Nevertheless, the present results provide a good working hypothesis based on the data that is currently available. Indeed, this impact of volcanic eruptions explains several aspects of recent AMOC variations, and associated patterns (for example, GSAs). Moreover recent analysis of the observed variability mode of bidecadal sea level reveals a strong regime shift since the 1970s [14] , which can be related to the ocean circulation changes described here in response to the Agung eruption. Nevertheless, processes other than volcanic eruptions may have shaped variability in the North Atlantic over the last six decades, such as the NAO ( Fig. 8 ) or the 1980s GSA, which is not attributed here to volcanic eruptions. We also stress the fact that the proposed mechanisms identified in the IPSL-CM5A-LR simulations are not at play for eruptions with a radiative forcing 50% larger than that of Agung (see for example, Supplementary Fig. 11 ). Different ranges of the sea-ice response [34] can indeed either increase or decrease convection, depending on the size of the eruption. This sensitivity to volcanic forcing is therefore expected to be model dependent and other models from our Bi-Dec ensemble may exhibit different thresholds and sensitivity to volcanic eruption size. Further analysis of this sensitivity is necessary to improve our understanding of the response of the climate system to volcanic eruptions, within a coordinated intercomparison framework. This will hopefully be implemented within the CMIP6 framework in the near future. The present findings also imply a significant predictability of the North Atlantic dynamics if an Agung- or Pinatubo-like eruption occurs in the future ( Fig. 9a ). Excited bidecadal variability would be superimposed on the long-term decreasing trend, which is driven by global warming [6] . Given the potential influence of AMOC and the North Atlantic Ocean on hurricane activity [58] , African Sahel drought [59] , Greenland melt [2] , regional sea level [60] and marine ecosystems, such decadal predictability is of key interest to a diversity of stakeholders, including the agriculture, energy, fisheries, insurance industries, water supply and management agencies. CMIP5 analysis We use the CMIP5 database of historical simulations for the period 1850–2005 ( http://cmip-pcmdi.llnl.gov/cmip5/ ), performed using solar, volcanic and anthropogenic forcings, and pre-industrial control simulations, performed without changes in forcing, to explore the variability of the simulated subpolar AMOC. This analysis is restricted to the 19 models for which the meridional stream function output is available ( Supplementary Table 1 ). Based on the information from several paleoclimate archives from the North Atlantic, which consistently show bidecadal variability (see main text), we select the subset of models for which a peak of energy significantly larger than a red noise process is present in the spectral band of 10 to 30 years. A power spectrum analysis ( Supplementary Fig. 1 ) is used to identify this subset of models for which spectral power is expressed in the 10–30-year period band, and passes a significance test (that is, the one that refutes the red noise null hypothesis) in either the pre-industrial or historical simulations. Almost half of the CMIP5 climate models (9 among 19 models) do satisfy this criterion: CCSM4, CESM1-BGC, MRI-ESM, NorESM1-ME, NorESM1-M, CanESM2, GFDL-ESM2M, GFDL-CM3 and IPSL-CM5A-LR. Supplementary Table 1 summarizes the main findings in terms of spectral characteristics of the AMOC at 48°N in the different models and simulations. Supplementary Figure 2 shows the AMOC evolution from some of the selected models over the period 1950–2005. These models show relatively well-phased variability close to harmonic variations with a maximum in the late 1970s and another one in the late 1990s. This extends the findings of Swingedouw et al . [15] using the IPSL-CM5A-LR model. Supplementary Figure 5 illustrates the phasing in terms of salinity and temperature, averaged in the upper Labrador Sea, found in these models IPSL-CM5A-LR simulations The ocean-atmosphere coupled model mainly used in this study is the IPSL-CM5A (ref. 36 ) in its low-resolution (LR) version as developed for CMIP5. The atmospheric model is LMDZ5 (ref. 61 ) with a 96 × 96 × L39 regular grid and the oceanic model is NEMO [62] with an 182 × 149 × L31 non-regular grid, in version 3.2, including the LIM-2 sea ice model [63] and the PISCES [51] module for oceanic biogeochemistry. The internal variability of the AMOC has been described in the study by Escudier et al . [20] It has a 20-year preferential variability in the whole subpolar gyre. The mechanism explaining such a variability was shown to be a cycle beginning (for instance) with an intensification of the EGC that brings more cold and fresh water to the Labrador Sea where it accumulates and gives rise to negative SST and sea surface salinity (SSS) anomalies. These anomalies are advected along the subpolar gyre; they affect the convection all along their path up to the Nordics Seas, where the negative SST anomalies increase the sea-ice cover, which in turn induces a positive sea-level pressure anomaly and a localized anticyclonic atmospheric circulation. This leads to a decrease in the wind stress along the eastern coast of Greenland and thus a weakening of the EGC, leading to an opposite phase of the cycle around 10 years after its onset. This cycle impacts the AMOC variations through the contribution of SSS anomalies to the convective activity in the subpolar North Atlantic. The list of simulations performed with this model and used in this study is summarized in the Supplementary Table 2 and described below. The five-member ensemble of historical simulations use a prescribed external radiative forcing from the observed increase in greenhouse gases and aerosol concentrations as well as the ozone changes ( Fig. 1 ) and the land-use modifications (not shown, see the study by Dufresne et al . [36] ). They also include estimates of solar irradiance variations and of volcanic eruptions over the historical period represented as a decrease in the total solar irradiance (depending on the intensity of the volcanic eruption, Fig. 1 ). These historical simulations start from year 1850. Their initial conditions come from different dates of the 1000-year control simulation under pre-industrial conditions, each separated by 10 years. This control pre-industrial simulation is itself starting after thousands of years of spin-up procedure. To evaluate the hypothesis of a destructive interference due to the Pinatubo eruption, we prepared an additional five-member ensemble using the IPSL-CM5A-LR model. The simulations start on 1 January 1991 from each historical simulation described earlier. They use rigorously the same external forcing except for the effect of the Pinatubo eruption, which was removed from the total solar irradiance. The AMOC response with the s.d. of the ensemble is shown in Supplementary Fig. 10 . We also consider a five-member ensemble of nudged simulations, for which each simulation includes a nudging term towards observed anomalous monthly SST (ref. 15 ). Each simulation starts on 1 January 1949 from one of the historical simulations presented above. These nudged simulations are using the same external forcing as the historical ones ( Fig. 1 ). The nudging technique consists in adding a heat flux term Q to the SST equation under the form Q=−κ ( SST ′ mod —SST ′ obs ) where SST ′ mod stands for the modelled anomalous SST at each time step and grid point, and SST ′ obs the anomalous observed SST (Reynolds et al . (2007)). Anomalies are computed with respect to the average SST over the period 1949–2005 in the corresponding historical simulation and in the observations. We use a restoring coefficient κ of 40 W m −2 K −1 corresponding to a relaxing time scale of ~60 days (for a mixed layer of 50 m depth). See the study by Swingedouw et al . [15] for further details. The CMIP5 last millennium simulation starts in 850. It includes solar [64] and volcanic forcing [53] . The implementation of the volcanic forcing in this simulation is slightly different from that used for the historical simulations. In the latter, the effect of stratospheric injection of sulphate volcanic aerosols is only considered as a modulation in the total solar irradiance variations, while in this simulation the volcanic aerosols in the stratosphere are transported latitudinally in the model following Grieser and Schonwiese [65] parameterization. We consider 48 latitude bands for this transport. The model uses prescribed changes in aerosols optical depth and interactively computes the perturbed (longwave and shortwave) radiative budgets. The reconstruction of aerosols optical depth uses sulphate data from ice cores records from Greenland and Antarctica [53] . In this simulation, the AMOC at 48°N shows very strong variability in the bidecadal band ( Supplementary Fig. 6 ), as in pre-industrial simulations analyzed in the study by Escudier et al . [20] and in the historical simulations ( Supplementary Fig. 1 ). For the analysis of the Agung-like eruptions, we consider the 40 years following each selected event as an individual sensitivity experiment, like the member of an ensemble. The selected volcanoes are shown with respect to the full time series of volcanic forcing over the last millennium in Supplementary Fig. 7 . The ensemble mean and the s.d. of the five members are shown in Fig. 3 . We only consider eruptions with a magnitude comparable to Agung (1963), since larger eruptions lead to very strong cooling resulting in a different regime response for the AMOC [34] . Note that although the selection of the individual volcanic events includes a condition on the absence of significant eruption during the 40 years after the event, no condition is imposed regarding the years preceding the selected eruption. It is nevertheless possible that volcanic eruptions occurring a few years earlier could also impact North Atlantic variability, and indeed it is possible that the 1460 eruption is affected in this way, although none of the other volcanoes selected. Since removing this eruption does not modify the main conclusions, we keep it in our pool. Sensitivity of IPSL simulations to the size of eruptions Our analyses are focused on the model response to moderate eruptions. Indeed, a composite computation of key oceanic variables in the North Atlantic for all volcanoes lower than one and a half Agung as shown in Supplementary Fig. 11 for the IPSL-CM5A-LR model clearly supports our results: this shows again that moderate-size volcanic eruptions excite the 20-year variability through a cooling of the Nordic Seas at lag 1 year, when the subpolar region is less affected. This leads in the following years to the build-up of SST positive anomalies (as well as SSS, not shown) in the Labrador Sea, which are then advected along the subpolar gyre affecting the mixed layer depth around lag 5–6 years, explaining the 15-year lag for maximum AMOC following the simple scheme from the study by Escudier et al . [20] However, volcanic eruptions larger than one and half Agung have a direct negative impact on SST in the convection region south of Iceland, leading almost immediately to local negative mixed layer depth anomalies for lags 2–6 years ( Supplementary Fig. 11 ) following the eruption onset, which will lead to AMOC weakening around year 9–13, consistent with the study by Mignot et al . [34] Such sensitivity could clearly be model dependent, so that further analysis of different models will be necessary to exactly evaluate the volcanic eruption size that lead to different regimes in different models and in reality. Salinity data Observational salinity data have been downloaded from the Bedford Institute of Oceanography website ( http://www.bio.gc.ca/science/data-donnees/base/start-commencer-eng.php ). Their analysis is focused on the Labrador Sea area, which is a key for the processes involved in the 20-year variability [20] . Since changes in deep convection driving the AMOC can be triggered by salinity anomalies in the Labrador Sea as deep as 300 m, we also consider subsurface data to this depth [20] . To evaluate the observational uncertainty, we also use the version 2a of data compilation from EN3 ( http://www.metoffice.gov.uk/hadobs/en3 ), and a SSS data compilation from ships of opportunity and oceanographic cruises [42] for the eastern part of the subpolar gyre. In situ temperature anomalies In the IPSL-CM5A-LR climate model, the salinity anomalies are associated with temperature anomalies in the Labrador Sea and all along the subpolar gyre and Nordic Seas [20] . This is related to variations of the EGC, which brings cold and fresh water from the Arctic. We check in Supplementary Fig. 4 that, in the data analyzed, the salinity anomalies shown in Fig. 2 have a temperature counterpart (using the same source of data, that is, Bedford Institute of Oceanography and EN3). It is clearly the case in the Labrador Sea, with once again an agreement between historical simulations and temperature data, following the GSAs of the 1970 and 1990s. We note that the GSA of the 1980s is not clear in the Bedford Institute of Oceanography data set and absent in the model. We argue that this GSA is primarily driven by exceptional atmospheric forcing [22] . Given the lack of strong signals in the eastern subpolar gyre, the correspondence between temperature and salinity anomalies is weaker in this area. Greenland ice core composite The δ 18 O Greenland records used herein correspond to six annually resolved millennial-long ice core records covering the period 1000–1973 (B18, Crete, DYE-3, GISP2, GRIP, NGRIP, see for example, Supplementary Table 3 ). During the instrumental period, the first PC associated with the leading EOF of these proxies (accounting for 25% of the variance of the six ice core records) is closely related to precipitation-weighted Greenland surface temperature changes [66] , ultimately driven by changes in the four major weather regimes in the North Atlantic, namely the two phases of the NAO, the Atlantic Ridge and the Scandinavian Blocking [66] . Our PC is closely related, during the overlapping period, ( R =0.67, P <0.05) to the average of five Arctic and Greenland δ 18 O ice core records previously used to characterize the bidecadal SST variability in the North Atlantic during the past 700 years [16] . Bivalve proxy records The bivalve data used are described in the study by Butler et al . [49] This proxy is a unique record of bivalve growth north of Iceland, annually resolved over a period of 1,357 years. Radiocarbon measurements taken on absolutely dated shell material have been used to show the co-varying influence of Atlantic and Arctic waters on the North Icelandic Shelf over the past millennium [67] . The correlation between growth and observed temperature is positive and weak (0.217, P <0.05 using HadISST1 gridded data), suggesting that the bivalves are responding to a nutrient signal that is only partially temperature driven. Link between last millennium proxies and model simulation The AMO [45] represents the low-frequency variations of SST averaged over the Atlantic from the equator to 60°N. These multidecadal variations influence surrounding regions. In particular, Greenland climate is considered to be very sensitive to these variations. For instance, surface air temperature at Nuuk, West Greenland and the AMO Index are highly correlated ( r =0.49, P =0.05) over the last 150 years [68] . Last, we show that in IPSL-CM5A-LR (and other models) the AMOC is leading the AMO by a few years [41] . Here we focus on the link between the AMOC and the SST in the North Atlantic and investigate the phase lag in Supplementary Fig. 8 using 1,000 years of the last millennium simulation. We show that AMOC index at 48°N is leading the SST in the Atlantic between 25 and 55°N by around 5–10 years. This phasing also clearly appears in the 40 years following selected volcanic eruptions from Fig. 3 . Strong correlations are also identified for the control simulation under pre-industrial conditions, showing that this behaviour is not triggered by external forcing but is linked to the internal mechanisms relating AMOC and North Atlantic SST (not shown). Conceptual models We build here a family of simple conceptual models to capture the essence of the main mechanisms at play in our climate model and hopefully in reality. Our first assumption, suggested by our results from the different CMIP5 screened models and data sets, is that Pinatubo-like eruptions lead to an AMOC maximum around 15 years after the onset of the volcanic eruption. This delay is related to the characteristic time required for the North Atlantic to adjust to the volcanic signal, through induced changes in convection. It accounts for the lag between cooling of Nordic Seas, reductions in EGC, positive anomalies advected along the subpolar gyre, changes in convection sites and, a few years later, changes in the AMOC [15] . This AMOC response corresponds to the excitation of damped oscillatory variations with a typical time scale of 20 years [69] . We call τ the time delay for a particular volcanic eruption to have an impact on the AMOC; it is expected to depend on the typical 15-year delay as well as on the exact timing of the eruption. The subsequent damped oscillation response excited by the volcano can then be described through the following function of time f ( t ): where H stands for the Heaviside function, t is the time and Δ is a characteristic damping time scale. Over the time period 1960–2010, there have been three main eruptions (Agung, El Chichon and Pinatubo) whose radiative forcing in the IPSL-CM5A-LR historical simulations are 1.5 W m −2 , 1.2 W m −2 and 2.1 W m −2 , respectively ( Fig. 1 ). To account for the size of the eruption, we introduce a scaling factor λ i for each volcano (equal to its radiative forcing). We finally use a factor α to scale globally the effect from all the volcanoes. For comparison with historical simulations and projections, we must also take into account the AMOC decreasing trend produced in response to anthropogenic forcing by CMIP5 models [6] . This effect of global warming is implemented through the GW( t ) function, which corresponds to the anthropogenic radiative forcing multiplied by a scaling factor β . This conceptual model can be tested with and without the Pinatubo eruption. When excluding the Pinatubo eruption, the sum in equation (2) only accounts for the two other volcanoes, and the rest stays the same. In reality, AMOC is also affected by the internal variability of the atmospheric circulation and is particularly sensitive to the NAO [3] , [55] , [56] with a 5-year lag. To include this aspect in the conceptual model, an additional term is introduced. It corresponds to the winter NAO index from NOAA ( http://www.cpc.ncep.noaa.gov/products/precip/CWlink/pna/JFM_season_nao_index.shtml ), with a lag of 5 years, due to oceanic adjustment to changes in surface fluxes and scaled by a coefficient γ. The tuning of the adjustable parameters of this conceptual model ( α , β , Δ and γ ) is performed with a minimization technique using IPSL-CM5A-LR simulations as targets. The global warming scaling β is first adjusted using all IPSL-CM5A-LR available projections. A linear regression performed between anthropogenic forcing and the simulated 48°N AMOC index leads to a scaling factor β of 1.2 Sv m 2 W −1 . We then define a cost function to be minimized, as the mean squared error between the conceptual model results and the reference simulation (historical and sensitivity experiments without Pinatubo eruption) over the period 1975–2030 ( Supplementary Fig. 12 ). The best choice for the scaling factor α for the volcanoes and the damping factor Δ for the oscillations is unequivocally 0.5 Sv and 60 years, respectively. Finally, the scaling factor γ for the NAO-forced AMOC variations is adjusted using the IPSL-CM5A-LR nudged simulations towards observed SST and optimized for a value of 2.5 Sv. We compare the results of two different conceptual models, which account for volcanic-induced variability and NAO forcing. Indeed, between 1975 and 2010, the volcanic excitations of the bidecadal mode acts on the timing of decadal variations; however, NAO is the main driver of the magnitude of AMOC variations in the conceptual model scaled on IPSL-CM5A-LR simulations ( Fig. 9c ). Indeed, if we compute the ratio of variance between the different conceptual models ( Fig. 9c ), including different pieces of forcing of the AMOC, we find that NAO alone accounts for 57% of the variance of the model including all processes, while the excitation of the bidecadal model accounts for 20%. Given that for any X and Y random variables, we have: Var( X+Y )=Var( X )+Var( Y ) +Cov ( X,Y ) where Var() is the variance operator and Cov() the covariance one. The sum of the variance explained by NAO and by volcanic-induced variability is not 100%, due to covariance. To avoid accounting twice for the role of volcanic eruption (through the radiative forcing and through the potential consequence on the subsequent winter NAO phase [27] ), we consider an alternative conceptual model, in which we remove the NAO forcing in the three winters following each eruption. In this case, the variance ratio between the variance of AMOC volcanically induced and the variance of AMOC, which is purely induced by the NAO (removing the three years following volcanic eruptions), is 30% and only 44% for the pure NAO-forced AMOC with volcanic years removed, respectively ( Fig. 9c ). The conceptual model is finally used to explore the impact of a hypothetical Pinatubo-like eruption starting in 2015 ( Fig. 9a ). Without such an event, and without large NAO changes, the conceptual model simulates only the gradual decreasing trend driven by global warming. If a large eruption were to occur in 2015, then it would excite large AMOC decadal oscillations with maximum strength in 2030 and minimum strength in 2040, potentially complicating the detection of long-term trends associated with global warming. How to cite this article: Swingedouw, D. et al . Bidecadal North Atlantic ocean circulation variability controlled by timing of volcanic eruptions. Nat. Commun. 6:6545 doi: 10.1038/ncomms7545 (2015).